Plasmon transport in graphene investigated by time-resolved electrical measurements Plasmons, which are collective charge oscillations, could provide a means of confining electromagnetic field to nanoscale structures. Recently, plasmonics using graphene have attracted interest, particularly because of the tunable plasmon dispersion, which will be useful for tunable frequency in cavity applications. However, the carrier density dependence of the dispersion is weak (proportional to n 1/4 ) and it is difficult to tune the frequency over orders of magnitude. Here, by exploiting electronic excitation and detection, we carry out time-resolved measurements of a charge pulse travelling in a plasmon mode in graphene corresponding to the gigahertz range. We demonstrate that the plasmon velocity can be changed over two orders of magnitude by applying a magnetic field B and by screening the plasmon electric field with a gate metal; at high B , edge magnetoplasmons, which are plasmons localized at the sample edge, are formed and their velocity depends on B , n and the gate screening effect. On metal surfaces, resonant interactions between electrons in nanoparticles and the electromagnetic field of light create surface plasmons. As the wavelength of surface plasmons can be reduced to the dimensions of electronic devices, plasmonics has been proposed to merge optics and electronics [1] , [2] , [3] . However, there is a fundamental limitation to using metals for plasmonics: plasmon properties cannot be altered once the material and the device geometry are fixed. In graphene, on the other hand, properties of sheet plasmons can be modified by electric-field doping [4] , [5] , [6] , [7] . The dispersion of sheet plasmons has been predicted to depend on the carrier density n , with the velocity varying as n 1/4 (ref. 6 ), which has recently been confirmed by the tunable resonant frequency in micro-ribbon structures [8] and optical nano-imaging [9] , [10] . Properties of plasmons in graphene can also be modified by applying a magnetic field B , which is manifested by the B -dependent resonance frequency of edge magnetoplasmons (EMPs) [11] in a cavity structure [12] . Here, we investigate plasmon transport in graphene in the time domain over a wide range of n and B by electrical time-of-flight measurements. To be specific, we measure the plasmon velocity through the time of flight of a pulsed charge generated by a voltage step applied to a gate electrode and travelling as a wave packet in the plasmon mode. We demonstrate that the measured velocity, which corresponds to the slope of the dispersion in the long-wavelength regime, can be tuned over two orders of magnitude between 10 4 and 10 6 m s −1 . In the absence of B , the velocity is higher than the Fermi velocity v F ~10 6 m s −1 , evidence for the transport of sheet plasmons. In the quantum Hall (QH) effect regime at high B , the plasmon transport is chiral and the velocity varies primarily reflecting the Hall conductance σ xy , indicating the formation of EMPs. In a sample with a metal gate, the velocity of EMPs is reduced by one order of magnitude and oscillates as a function of the Landau level filling factor ν . The wide tunability of the plasmon velocity through B , n and the gate screening effect encourages designing graphene nanostructures for plasmonic circuits [13] , [14] . Time-resolved measurement of plasmon transport For our time-resolved measurements, large-area graphene is essential for the time of flight to be long enough so that it can be resolved by electrical means. We prepared graphene on the Si-face of 4H-SiC ( Fig. 1a ) by thermal decomposition [15] . The surface of the devices was covered with 100-nm-thick hydrogen silsequioxane (HSQ) and 40-nm-thick SiO 2 insulating layers. As a result of n-doping from the interfacial buffer layer and p-doping from the HSQ layer, graphene has n-type carriers. Longitudinal R xx and Hall R xy resistances in a millimeter-scale Hall bar show well-developed ν =2 and 6 QH states ( Fig. 1b ), demonstrating that the carrier density is almost uniform on a large scale. 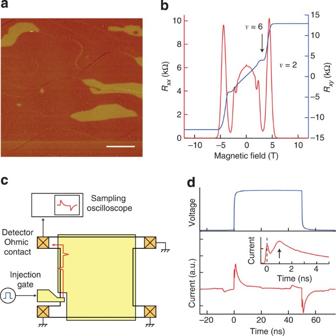Figure 1: Graphene on SiC and the experimental techniques. (a) Atomic force microscopy phase image of graphene on SiC (ref.27). Scale bar, 1 μm. Single-layer graphene (brown colour in majority regions) covers the substrate, while two or more graphene layers (yellow colour in minority regions) are formed along the terrace edge. As few-layer graphene regions are fragmented, the single-layer graphene dominates carrier transport. (b)RxxandRxyat 1.5 K of a Hall bar device with the channel width and length of 0.2 and 1.1 mm, respectively. The mobility is 12,000 cm2V−1s−1. (c) Schematic illustration (not to scale) of the sample structure and the experimental setup for the time-resolved transport measurement. (d) Voltage step with the height of 1 V and the time width of 50 ns applied to the injection gate (top) and temporal traces of the current detected by a sampling oscilloscope (bottom). The current is averaged over a few seconds on the period of the excitation voltage step. Small features around −10 and 40 ns are due to reflections in high-frequency lines. Inset shows the magnified view of the current trace aroundt=0. The sharp peak att=0 is due to direct cross-talk between high-frequency lines. The broad peak indicated by an arrow is due to the charge pulse arriving at the detector Ohmic contact. Figure 1: Graphene on SiC and the experimental techniques. ( a ) Atomic force microscopy phase image of graphene on SiC (ref. 27 ). Scale bar, 1 μm. Single-layer graphene (brown colour in majority regions) covers the substrate, while two or more graphene layers (yellow colour in minority regions) are formed along the terrace edge. As few-layer graphene regions are fragmented, the single-layer graphene dominates carrier transport. ( b ) R xx and R xy at 1.5 K of a Hall bar device with the channel width and length of 0.2 and 1.1 mm, respectively. The mobility is 12,000 cm 2 V −1 s −1 . ( c ) Schematic illustration (not to scale) of the sample structure and the experimental setup for the time-resolved transport measurement. ( d ) Voltage step with the height of 1 V and the time width of 50 ns applied to the injection gate (top) and temporal traces of the current detected by a sampling oscilloscope (bottom). The current is averaged over a few seconds on the period of the excitation voltage step. Small features around −10 and 40 ns are due to reflections in high-frequency lines. Inset shows the magnified view of the current trace around t =0. The sharp peak at t =0 is due to direct cross-talk between high-frequency lines. The broad peak indicated by an arrow is due to the charge pulse arriving at the detector Ohmic contact. Full size image For the time-resolved transport measurement, a pulsed charge is generated in graphene by applying a voltage step to the injection gate deposited across the sample edge ( Fig. 1c ): at the rising (falling) edge of the voltage step, a pulse of positive (negative) charges is induced through the capacitive coupling between the gate and graphene ( Fig. 1d ). The charge pulse propagates in graphene as a wave packet of a plasmon mode and is detected as a time-dependent current through the detector Ohmic contact using a sampling oscilloscope. We note that such time-domain measurements have been widely used to study EMPs in conventional two-dimensional electron systems (2DESs; refs 16 , 17 , 18 ) and are known to give a velocity consistent with frequency-domain measurements [19] , [20] . The detected current comprises two components, a sharp peak due to direct cross-talk between high-frequency lines and a broad peak that appears with a delay; the latter, which is due to the charge pulse arriving at the detector Ohmic contact, is the signal of our interest (inset of Fig. 1d ). As the cross-talk propagates with the speed of light and appears with virtually zero time delay, we set the origin of the time t =0 at the peak of the cross-talk. By analyzing the time profile of the broad peak, time of flight of charges is obtained. In all the measurements presented in this paper, a 100-ps rise time filter was used for the injection line to minimize the cross-talk. As the −3 dB band width of the rise time filter is 3.5 GHz, the frequency of plasmons should distribute below 3.5 GHz (Methods and Supplementary Fig. S1 ). We used two samples, one with and the other without a large top gate ( Fig. 1c ). In the ungated sample, the electron density is n =5 × 10 11 cm −2 , whereas in the gated sample n =1.2 × 10 12 cm −2 for a top gate bias V tg =0 V. In the ungated sample, the path length between the injection gate and the detector Ohmic contact is 1.1 mm. In the gated sample, the path length in the gated region is 0.2 mm. 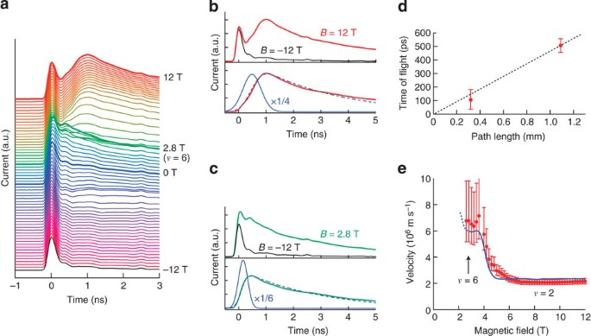Figure 2: Results of the time-resolved transport measurement for the graphene device without a top gate. (a) Current as a function of time around the positive charge transport for several magnetic fields betweenB=−12 (bottom) and 12 T (top). The path length between the injection gate and the detector Ohmic contact is 1.1 mm. The sign ofBis defined as positive whenBis applied from the back of the sample. Traces are vertically offset for clarity. (b,c), Examples for the data analysis. By subtracting the current trace atB=−12 T (black trace in the top panels) from that at eachB, cross-talk can be eliminated (red and green traces in the bottom panels ofbandc, respectively). The dashed traces are the results of fitting by the convolution of a Gaussian function and exp(−t/TRC) withTRC=3 ns. From the peak position of the Gaussian function (blue solid traces), the time of flight of the charge pulse is obtained. (d) We also obtained the time of flight atB=12 T in a sample with shorter path length of 320 μm. As expected, the time of flight is proportional to the path length. (e) Red circles are the velocity of the charge pulse determined from the time of flight. Blue line represents the velocity calculated using equation 1. For the calculation, we usedσxymeasured using the Hall bar sample. The size of the error bars originates from possible fluctuations in the cross-talk that may be induced by thermal drift or mechanical vibration of the high-frequency lines and/or magnetic field. We assumed that the amplitude of the cross-talk weakly fluctuates by 10%, which results in the uncertainty in the shape of the current traces to be fitted. All measurements were performed at 1.5 K. Plasmon velocity in the ungated sample Figure 2a shows the current traces for the sample without a top gate measured at various magnetic fields from −12 to 12 T. As expected for cross-talk, the sharp peak at t =0 is independent of B ; both its position and amplitude remain unchanged. Note that the ripples at t >0, which are also independent of B , are due to cross-talk that occurs through multiple reflections in the high-frequency lines. In contrast, the amplitude of the broad peak is strongly asymmetric with respect to the sign of B , indicating the chirality of the edge current: when B is applied from the back of the sample ( B >0), the chirality is clockwise and the injected charges travel to the detector Ohmic contact along the left edge ( Fig. 1c ); otherwise ( B <0), the charges flow to other grounded Ohmic contacts. For B >0, both the amplitude and the time delay of the broad peak vary with B . The amplitude is large around B =3 T and for B >5 T, where the ν =6 and ν =2 QH states are formed, respectively. This indicates that the charge relaxation is mainly due to scattering by electrons in bulk graphene. The delay time at the peak position is almost constant in the v =2 QH state for B >5 T. The delay time decreases with decreasing B and the peak is masked by the cross-talk for B <2.5 T. Figure 2: Results of the time-resolved transport measurement for the graphene device without a top gate. ( a ) Current as a function of time around the positive charge transport for several magnetic fields between B =−12 (bottom) and 12 T (top). The path length between the injection gate and the detector Ohmic contact is 1.1 mm. The sign of B is defined as positive when B is applied from the back of the sample. Traces are vertically offset for clarity. ( b , c ), Examples for the data analysis. By subtracting the current trace at B =−12 T (black trace in the top panels) from that at each B , cross-talk can be eliminated (red and green traces in the bottom panels of b and c , respectively). The dashed traces are the results of fitting by the convolution of a Gaussian function and exp(− t / T RC ) with T RC =3 ns. From the peak position of the Gaussian function (blue solid traces), the time of flight of the charge pulse is obtained. ( d ) We also obtained the time of flight at B =12 T in a sample with shorter path length of 320 μm. As expected, the time of flight is proportional to the path length. ( e ) Red circles are the velocity of the charge pulse determined from the time of flight. Blue line represents the velocity calculated using equation 1. For the calculation, we used σ xy measured using the Hall bar sample. The size of the error bars originates from possible fluctuations in the cross-talk that may be induced by thermal drift or mechanical vibration of the high-frequency lines and/or magnetic field. We assumed that the amplitude of the cross-talk weakly fluctuates by 10%, which results in the uncertainty in the shape of the current traces to be fitted. Full size image In our experiment, the width of the injected charge pulse is estimated to be 100 ps, which corresponds to the rise time of the excitation voltage step. The detected signal is much broader, with a long exponential tail whose decay time is almost independent of B . This is due to the RC time constant T RC =3 ns of the detector circuit arising from the contact resistance and stray capacitance (Methods and Supplementary Fig. S2 ). Figure 2b explains how to restore the waveform of the charge pulse and derive the time of flight from the measured current traces. First, we subtract the cross-talk from the measured current traces by regarding the B =−12 T trace (black traces in the top panel of Fig. 2b ) as representing the cross-talk waveform. Then we approximate the waveform of the charge pulse with a Gaussian and calculate its convolution with the response function exp( −t/T RC ). By using the height, width and the position of the Gaussian function as adjustable parameters, we can fit the convolution function to the current traces obtained by subtracting the cross-talk (bottom panel of Fig. 2b ). The extracted Gaussian width is of several hundred picoseconds, which is still several times larger than the width of the injected pulse, indicating that the charge pulse is broadened during the propagation, presumably by scattering and/or nonlinear dispersion. The time of flight of the charge pulse is obtained from the peak position of the Gaussian. To support the validity of our analyses, we carried out similar measurements using a sample with a shorter path length of 0.3 mm and found that the time of flight becomes smaller as expected ( Fig. 2d and Supplementary Fig. S3 ). The velocity of the charge pulse determined from the time of flight and the path length depends on B ( Fig. 2e ). It is almost constant at about 2 × 10 6 m s −1 in the ν =2 QH state. As B is decreased, the velocity increases and shows a plateau at 6 × 10 6 m s −1 for the ν =6 QH state. For smaller B , the velocity cannot be determined accurately because the broad peak largely overlaps with the cross-talk around t =0. This indicates that the charge velocity for smaller B is above the maximum measurable value of 6 × 10 6 m s −1 , which is larger than v F ~10 6 m s −1 ( Supplementary Fig. S4 ). This demonstrates that the charge pulse propagates not as individual electrons but as collective modes, that is, plasmons. This is consistent with sheet-plasmon theory for low-frequency limit [6] . The plateau structures in the velocity for the ν =2 and 6 QH states suggest that the velocity is primarily a function of σ xy . This feature is an indicator of EMPs [11] , [21] . We analyse the velocity for higher B based on the theory for EMPs in a standard 2DES. For an ungated 2DES with a hard-wall edge potential, the velocity of EMPs is given by [11] where is the dielectric constant; we used , which is the average of the values of the HSQ insulating layer and the SiC substrate . w is the transverse width of EMPs given by , reflecting the ratio of the Coulomb energy to the cyclotron energy [11] . Here, m is the effective mass, for which we take the cyclotron mass . Then, w is calculated to be 5.2 nm at B =12 T and increases with decreasing B ; as n in graphene on SiC depends on the Fermi energy, we calculate it using the measured R xy (refs 22 , 23 ). The value of k relevant to the experiment can be crudely estimated from the time width of the plasmon pulse obtained by the convolution fitting ( Fig. 2b ). The time width, together with the velocity measured at each B , translates into a spatial width of the pulse, which provides k ~10 4 m −1 as a lower bound. Note that k dependence of the EMP velocity is weak, e.g., when k is increased by a factor of 10, the velocity decreases only by 30%. Without any fitting parameter, the experimental result can be well reproduced by equation 1. For B <2 T, the condition σ xx < σ xy ( σ xx : diagonal conductivity), necessary for equation 1 to be applicable, no longer holds. The good agreement between experiment and theory at high B indicates that charge excitations in graphene propagate in the form of EMPs with a hard-wall edge potential. Plasmon velocity in the gated sample In a gated sample, the electric field accompanying plasmons is screened by the gate metal. The degree of the screening can be represented by the ratio w/d , where d =140 nm is the distance between graphene and the gate metal. Therefore, by varying w through n and B , the screening effect can be examined. 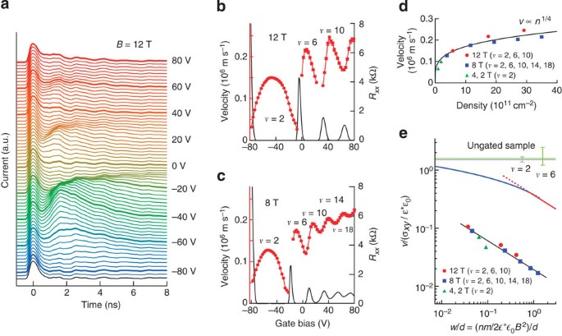Figure 3: Results of the time-resolved transport measurement for the graphene device with a top gate. (a) Current as a function of time atB=12 T for several values ofVtg. Traces are vertically offset for clarity. The charge neutrality point is located atVtg=−85 V and the electron density increases withVtg. (b,c) Velocity of the charge pulse in the gated region forB=12 and 8 T. The path length is 0.2 mm. Black traces representRxx. (d) Velocity at peaks in QH states plotted as a function of the carrier density. In addition to the data points taken frombandc, those forν=2 atB=4 and 2 T are included. The solid curve representsvn1/4. (e) Log–log plot of the velocity at peaks normalized byas a function ofw/d, where. Solid black line is. Blue and red curves are the normalized velocity calculated by using equations 2 and 3, respectively. Grey and green lines with an error bar represents the normalized velocity atν=2 and 6 in the ungated sample, respectively. Figure 3 shows results for the sample with a top gate. In Fig. 3a , the current traces at B =12 T for various values of V tg are plotted. At V tg =−85 V (bottom trace), the system is at the charge neutrality point, where the signal due to plasmons is absent; by subtracting the current trace at V tg =−85 V from that for each V tg , direct cross-talk at t =0 and cross-talk with finite delay due to multiple reflections can be eliminated. As V tg is increased, the signal becomes large in the QH states at . The time of flight oscillates as a function of the filling factor. Note that we measured the time of flight in a sample with the path length of 0.8 mm, in addition to that of 0.2 mm, and confirmed that the time of flight varies with the path length ( Supplementary Fig. S3 ). Similar measurements were carried out at several magnetic fields, and the velocity at B =12 and 8 T is plotted in Fig. 3b , respectively, as a function of V tg . The velocity oscillates with peak values around 2 × 10 5 m s −1 in QH states; these values are one order of magnitude smaller than that in the ungated sample. The velocity oscillation can be explained in terms of the ν -dependence of dissipation. Theory shows that dissipation not only damps EMPs but also slows them down [24] : in QH states (where ), dissipation becomes minimum and thus the velocity becomes maximum ( Supplementary Figs S5,S6 ). Figure 3: Results of the time-resolved transport measurement for the graphene device with a top gate. ( a ) Current as a function of time at B =12 T for several values of V tg . Traces are vertically offset for clarity. The charge neutrality point is located at V tg =−85 V and the electron density increases with V tg . ( b , c ) Velocity of the charge pulse in the gated region for B =12 and 8 T. The path length is 0.2 mm. Black traces represent R xx . ( d ) Velocity at peaks in QH states plotted as a function of the carrier density. In addition to the data points taken from b and c , those for ν =2 at B =4 and 2 T are included. The solid curve represents v n 1/4 . ( e ) Log–log plot of the velocity at peaks normalized by as a function of w/d , where . Solid black line is . Blue and red curves are the normalized velocity calculated by using equations 2 and 3, respectively. Grey and green lines with an error bar represents the normalized velocity at ν =2 and 6 in the ungated sample, respectively. Full size image Here, we focus on the velocity at peaks, where the effects of dissipation become minimal, and examine the gate screening effect. We analyse the data using an EMP theory developed for a standard 2DES. For a gated 2DES with a hard-wall edge potential, the velocity can be expressed as a function of w / d in the following two forms sharing the prefactor (ref. 11 ), Which functional form applies depends on the range of the parameter w / d . In Fig. 3e , we show the measured velocity normalized by as a function of w / d for comparison with equations 2 and 3; to match the velocity calculated using the two equations at w = d , the value calculated with equation 3 is multiplied by a factor of 0.53. For the plot of the measured velocity, we estimated w using the relation based on the model in [11] . The values of the normalized velocity at ν =2 and 6 in the ungated sample are shown in grey and green lines as a reference for the weak-screening limit. Theoretically, the gate screening reduces the velocity by about one order of magnitude when . As w / d decreases, the effect of the gate screening weakens as , decreasing to a factor of two when . Experimentally, we find the gate screening effect to be much stronger than that predicted by the theory, reducing the velocity by one order of magnitude even when . Notably, the normalized velocity versus w / d follows a power law as . As σ xy n / B and w n 3/2 / B 2 , the power law implies v n 1/4 ( Fig. 3d ), exactly the carrier density dependence specific to sheet plasmons in graphene at B =0 T (refs 6 , 7 ). In the ungated sample, the plasmon velocity is of the order of 10 6 m s −1 and decreases with increasing B . This can be reproduced qualitatively and quantitatively by the theory for EMPs at a hard-wall edge potential. In the gated sample, the velocity is of the order of 10 5 m s −1 and decreased by the gate screening, following a power law . The effect of the gate screening is much stronger than that predicted by the theory for (equation 2), relevant to the experimental condition. Here, we note that the power law is just what is expected from equation 3 appropriate to . This would suggest that the actual width of EMPs is larger than the calculated w . If this is the case, the data in Fig. 3e should shift to the larger w / d side, which mitigates both qualitative and quantitative disagreement. As w depends on the dielectric environment near the graphene edge, it would be modified by the gate screening. For the full understanding, further experiments with controlled environment and theory specialized for graphene EMP, which takes account of the details of the dielectric environment, would be necessary. In summary, we have carried out time-of-flight measurements of plasmons in graphene. The plasmon velocity determined by the time of flight and the path length varies over two orders of magnitude between 10 4 and 10 6 m s −1 , depending on B , n , and the gate screening effect. The wide tunability of the plasmon velocity encourages designing graphene nanostructures for plasmonic circuits. During the preparation of the manuscript, we became aware of a related unpublished work [25] , which reports chiral EMPs in exfoliated graphene. Device fabrication We prepared a graphene wafer by thermal decomposition of a 4H-SiC(0001) substrate. SiC substrates were annealed at around 1,800 °C in Ar at a pressure of less than 100 Torr (ref. 15 ). For the fabrication of devices, graphene and the SiC were mesa-etched in a CF 4 atmosphere. After the etching, Cr/Au electrodes were deposited and then the surface was covered with 100-nm-thick HSQ and 40-nm-thick SiO 2 insulating layers. For the injection gate and the top gate, Cr/Au was deposited on the insulating layers. Although steps of the SiC substrate have been reported not to affect the plasmon dispersion [26] , to minimize this possible effect, the edge between the injection gate and the detector Ohmic contact is aligned parallel to the substrate steps. Injection and detection of plasmons We excited plasmons in graphene by applying a voltage step to the injection gate. High-frequency measurements are often affected by cross-talks. As the cross-talk is stronger for higher frequency, we attenuated high-frequency components in the excitation voltage step using a 100-ps rise time filter ( Supplementary Fig. S1 ). By comparing current traces taken with and without the filter, we confirmed that the filter strongly suppresses the cross-talk, while does not affect the signal associated with plasmons. Plasmons are detected as a time-dependent current through the detector Ohmic contact using a sampling oscilloscope. The time constant of the detection is estimated to be 3 ns ( Supplementary Fig. S2 ), determined by the RC time constant of the measurement system. The contact resistance in our graphene devices is as large as several kilo-ohms and, together with a stray capacitance, it forms a low-pass filter: when the contact resistance is kΩ, a reasonably small stray capacitance pF leads to ns. It should be noted that the time constant does not limit the time resolution of the time of flight. As shown in Fig. 2b , the waveform of the charge pulse can be obtained by the convolution fitting. Then the time resolution is limited by the width of the charge pulse. How to cite this article: Kumada, N. et al . Plasmon transport in graphene investigated by time-resolved electrical measurements. Nat. Commun. 4:1363 doi: 10.1038/ncomms2353 (2013).